SPEN is required forXistupregulation during initiation of X chromosome inactivation At initiation of X chromosome inactivation (XCI), Xist is monoallelically upregulated from the future inactive X (Xi) chromosome, overcoming repression by its antisense transcript Tsix . Xist recruits various chromatin remodelers, amongst them SPEN, which are involved in silencing of X-linked genes in cis and establishment of the Xi. Here, we show that SPEN plays an important role in initiation of XCI. Spen null female mouse embryonic stem cells (ESCs) are defective in Xist upregulation upon differentiation. We find that Xist -mediated SPEN recruitment to the Xi chromosome happens very early in XCI, and that SPEN-mediated silencing of the Tsix promoter is required for Xist upregulation. Accordingly, failed Xist upregulation in Spen −/− ESCs can be rescued by concomitant removal of Tsix . These findings indicate that SPEN is not only required for the establishment of the Xi, but is also crucial in initiation of the XCI process. To compensate for gene-dosage imbalance between females (XX) and males (XY), female placental mammals randomly inactivate one X chromosome early during embryonic development [1] . In mice, random X-chromosome inactivation (XCI) takes place in the epiblast in three phases: initiation, establishment, and maintenance. During the initiation phase, the long noncoding RNA (lncRNA) Xist is upregulated from the future inactive X (Xi) chromosome [2] , [3] , [4] . Xist is located within the X Chromosome Inactivation Centre ( Xic ), an X-linked region required for XCI that contains different cis -regulatory elements, including Tsix , another lncRNA gene that is transcribed antisense to and completely overlaps Xist [5] . Tsix negatively regulates Xist expression via antisense transcription and chromatin remodeling [6] , [7] , [8] , [9] , [10] , [11] , [12] . Together , Xist and Tsix form a master switch that controls initiation of XCI: in the pluripotent state, Tsix is biallelically expressed, repressing both alleles of Xist , while upon initiation of XCI, the balance changes, resulting in downregulation of Tsix and upregulation of Xist on the future Xi. Trans -regulators including pluripotency factors OCT4, NANOG, REX1 as well as XCI activators are key in controlling this switch by regulating Xist and Tsix transcription (reviewed in [13] ). Later, during the establishment phase of XCI, the 17 kb lncRNA Xist spreads in cis along the future Xi and recruits different proteins involved in gene silencing that render the X transcriptionally inactive (reviewed in [14] ). Active histone marks (H3K4me2/me3, H3 and H4 acetylation) are removed and repressive histone marks are instigated, catalyzed by polycomb group complexes and other protein complexes (reviewed in [15] ). Finally, in the maintenance phase, the inactive state of the Xi is epigenetically propagated across cell divisions. Different studies consisting of Xist RNA immunoprecipitations coupled to mass spectrometry [16] , [17] , [18] and genetic screens [19] , [20] identified SPEN (also known as SHARP in human and MINT in mouse) as a crucial factor in the establishment phase of XCI. SPEN is a large protein with four N-terminal RNA recognition motifs (RRM) and a highly conserved C-terminal SPOC domain able to recruit different proteins involved in transcriptional silencing [21] , [22] . SPEN is also involved in the Notch signaling pathway and nuclear receptor signaling, where it acts as a transcriptional corepressor [23] , [24] . SPEN is crucial for X-linked gene silencing [16] , [17] , [19] , [20] by binding the Xist repeat A (RepA) via its RRM domains [17] , [19] and interacting via its SPOC domain with the corepressors NCoR/SMRT to recruit/activate histone deacetylase 3 (HDAC3), responsible for the removal of histone H3 and H4 acetylation at promoters and enhancers of genes located on the future Xi [16] , [25] . 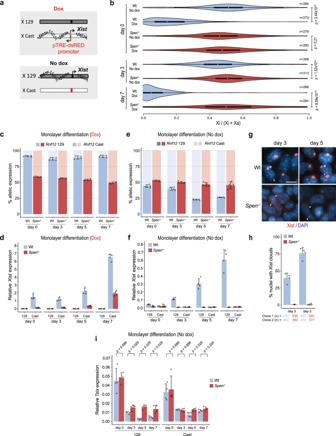Fig. 1: ImpairedXistupregulation inSpen−/−ESCs upon monolayer differentiation. aOverview of the endogenous doxycycline-inducibleXisthybrid system used in this study. Addition of doxycycline leads to inactivation of the Cast X chromosome, while no addition of the drug leads to inactivation of the 129 X chromosome.bViolin plots depicting the distribution of the allelic ratios ((Xi)/(Xi+Xa)) of X-linked genes in Wt andSpen−/−ESCs, untreated or treated with doxycycline at days 0, 3, and 7 of differentiation. This figure summarizes data in Supplementary Fig.1e. The box plots inside the violin plots display the median (central white dot), the interquartile range (box limits) and the whiskers represent 1.5x of the interquartile range. Two-sided Mann–Whitney test corrected with Benjamini–Hochberg for multiple testing (α < 0.05).n= genes with more than 20 reads. Xa = active X chromosome.cPercentage ofRnf12allelic expression at different time points of monolayer differentiation of two independent Wt andSpen−/−ESC lines treated with doxycycline, determined by RT-qPCR. RelativeRnf12allelic (129 and Cast) expression was normalized toRnf12total expression and averaged ± standard deviation (SD). Reference gene:Hist2h2aa1.dRelative allele-specificXistexpression of two independent Wt andSpen−/−ESC lines at different time points of monolayer differentiation treated with doxycycline. Average expression ± SD. Reference gene:Hist2h2aa1.eSame as displayed in (c) without doxycycline.fSame as displayed in (d) without doxycycline.gXistRNA FISH (red) of Wt andSpen−/−ESC lines at days 3 and 5 of differentiation. BothTsixpinpoints (arrowheads) andXistclouds (asterisks) are visible. DNA is stained with DAPI (blue). Scale bar: 10 µm.hQuantification of (g), displaying the average percentage of nuclei withXistclouds. Average percentage ± SD, the total number of counted nuclei per clone is indicated.iRelative allele-specificTsixexpression of Wt and Spen−/−ESCs at different time points of monolayer differentiation, determined by RT-qPCR. Average expression ± SD. Two-sided Mann–Whitney test (α< 0.05). Reference gene:Hist2h2aa1. (c–f, h, i)n= 4 biological replicates including 2 independent clones (squares vs. circles) per condition. Despite this crucial role for SPEN in establishment of the Xi, these studies did not report defects in Xist upregulation and coating [16] , [17] , [19] , [20] , [25] , possibly due to forced Xist upregulation using doxycycline-inducible systems (Supplementary Table 1 ). Here, we show that SPEN accumulates on the Xi very early during differentiation and is required for Xist upregulation. We show that SPEN has a dual function, required to silence Tsix and facilitate Xist upregulation, and stabilization of Xist RNA. Together, our results indicate that SPEN is not only necessary for X-linked gene silencing, but also plays a crucial earlier role in the regulation of initiation of XCI. SPEN is required for Xist upregulation Previous work has shown how SPEN is crucial for silencing of X-linked genes, but these studies did not investigate the role of SPEN in initiation of Xist expression. Therefore, we generated Spen homozygous ( Spen −/− ) and heterozygous ( Spen +/− ) knockout mouse embryonic stem cells (ESCs) by deleting the complete open-reading frame (ORF) using the CRISPR/Cas9 technology (Supplementary Fig. 1a ). These lines were generated in a hybrid F1 129/Sv:Cast/EiJ (129/Cast) genetic background with a doxycycline-responsive endogenous Xist promoter located on the Cast X chromosome [26] (Fig. 1a ). The S pen ORF deletion was verified by PCR on genomic DNA (gDNA) and Western blot analysis (Supplementary Fig. 1b,c ). Allele-specific RNA-seq analysis (Supplementary Fig. 1d ) of wild-type (Wt) undifferentiated ESCs (day 0) containing the doxycycline-responsive Xist promoter treated with and without doxycycline for 4 days showed skewed X-linked gene silencing toward the Cast allele (Fig. 1b , Supplementary Fig. 1e top left). On the other hand, the same analysis in Spen −/− ESCs showed impaired X-linked gene silencing (Fig. 1b , Supplementary Fig. 1e bottom left), as described before [16] , [17] , [19] , [20] (Supplementary Table 1 ). Fig. 1: Impaired Xist upregulation in Spen −/− ESCs upon monolayer differentiation. a Overview of the endogenous doxycycline-inducible Xist hybrid system used in this study. Addition of doxycycline leads to inactivation of the Cast X chromosome, while no addition of the drug leads to inactivation of the 129 X chromosome. b Violin plots depicting the distribution of the allelic ratios ((Xi)/(Xi+Xa)) of X-linked genes in Wt and Spen −/− ESCs, untreated or treated with doxycycline at days 0, 3, and 7 of differentiation. This figure summarizes data in Supplementary Fig. 1e . The box plots inside the violin plots display the median (central white dot), the interquartile range (box limits) and the whiskers represent 1.5x of the interquartile range. Two-sided Mann–Whitney test corrected with Benjamini–Hochberg for multiple testing (α < 0.05). n = genes with more than 20 reads. Xa = active X chromosome. c Percentage of Rnf12 allelic expression at different time points of monolayer differentiation of two independent Wt and Spen −/− ESC lines treated with doxycycline, determined by RT-qPCR. Relative Rnf12 allelic (129 and Cast) expression was normalized to Rnf12 total expression and averaged ± standard deviation (SD). Reference gene: Hist2h2aa1 . d Relative allele-specific Xist expression of two independent Wt and Spen −/− ESC lines at different time points of monolayer differentiation treated with doxycycline. Average expression ± SD. Reference gene: Hist2h2aa1 . e Same as displayed in ( c ) without doxycycline. f Same as displayed in ( d ) without doxycycline. g Xist RNA FISH (red) of Wt and Spen −/− ESC lines at days 3 and 5 of differentiation. Both Tsix pinpoints (arrowheads) and Xist clouds (asterisks) are visible. DNA is stained with DAPI (blue). Scale bar: 10 µm. h Quantification of ( g ), displaying the average percentage of nuclei with Xist clouds. Average percentage ± SD, the total number of counted nuclei per clone is indicated. i Relative allele-specific Tsix expression of Wt and Spen −/− ESCs at different time points of monolayer differentiation, determined by RT-qPCR. Average expression ± SD. Two-sided Mann–Whitney test ( α < 0.05). Reference gene: Hist2h2aa1 . ( c – f, h, i ) n = 4 biological replicates including 2 independent clones (squares vs. circles) per condition. Full size image To trigger XCI in the context of differentiation, we forced Xist upregulation by doxycycline treatment followed by monolayer differentiation. Allele-specific RNA-seq analysis of Wt and Spen −/− ESCs treated with doxycycline at day 7 of monolayer differentiation (Supplementary Fig. 1d ) also revealed a lack of X-linked gene silencing along the entire X chromosome (Fig. 1b , Supplementary Fig. 1e bottom right). Similarly, allele-specific RT-qPCR analysis of the X-linked gene Rnf12 revealed impaired silencing (Fig. 1c ). Although previous work indicated that in Spen −/− ESCs, a group of lowly expressed X-linked genes are susceptible to SPEN-independent gene silencing [27] , our RNA-seq analysis shows no silencing of this specific group of genes (Supplementary Fig. 1f,g ). We observed Xist upregulation in Wt and Spen −/− cells, however doxycycline induction resulted in lower Xist expression levels in Spen −/− compared with Wt ESCs (Fig. 1d ), an effect that was also reported in a recent study [27] . Next, we recapitulated physiological XCI by monolayer differentiation in the absence of doxycycline to allow normal Xist upregulation and X-linked gene silencing. Allele-specific RNA-seq analysis of Wt and Spen −/− ESCs at day 3 without doxycycline (Supplementary Fig. 1d ) shows a significant difference in silencing (Fig. 1b , Supplementary Fig. 1e top right) also visible for Rnf12 at day 3 by RT-qPCR and more pronounced at later time points of differentiation (days 5 and 7) (Fig. 1e ). Remarkably, in Spen −/− cells, Xist upregulation from the 129 allele was completely abrogated (Fig. 1f ), contrasting earlier evidence that suggested that SPEN is not required for Xist upregulation and coating [16] , [17] , [19] , [20] , [25] (Supplementary Table 1 ). In addition, differentiating Spen −/− ESCs lack Xist clouds, determined by RNA-FISH (Fig. 1g,h ), while Tsix was significantly more expressed from the Wt 129 allele in Spen −/− cells compared with Wt cells in differentiating cells (Fig. 1i ), suggesting that SPEN might be necessary for Tsix silencing. Importantly, RT-qPCR analysis confirmed proper silencing of pluripotency genes Rex1 and Nanog , and upregulation of endoderm marker Gata6 (Supplementary Fig. 1h ) in Spen −/− ESCs upon monolayer differentiation, indicating that loss of Xist expression is not related to defective ESC differentiation. Furthermore, while Spen +/− cells are able to upregulate Xist and silence Rnf12 upon doxycycline treatment followed by monolayer differentiation (Supplementary Fig. 2a,b ), they show reduced Rnf12 silencing upon physiological differentiation without a defect in Xist upregulation (Supplementary Fig. 2c,d ). Given that SPEN levels are reduced in Spen +/− cells (Supplementary Fig. 1c ), these results demonstrate that SPEN dosage is important in XCI. Spen rescue leads to normal Xist expression levels To confirm our results, we performed a rescue experiment by stably reexpressing Spen through introduction of the full-length Spen cDNA in the ROSA26 locus [25] of Spen −/− ESCs (Supplementary Fig. 3a ). Successful integration was verified by gDNA PCR and confirmed by Spen mRNA and protein levels by RT-qPCR and Western blot, respectively (Supplementary Fig. 3b–d ). The generated rescue clones (Clones A, B, and C) display two- to three-fold overexpression of Spen RNA at the ESC stage and during monolayer differentiation (Supplementary Fig. 3c ). In contrast to the Spen −/− lines, all Spen −/−(cDNA) rescue clones express Xist at similar levels to Wt clones during monolayer differentiation (Fig. 2a ). Allele-specific expression analysis of Rnf12 and Tsix (129 allele) indicated that the silencing defect is partially rescued in Spen −/−(cDNA) clones (Supplementary Fig. 3e, f ). Moreover, RT-qPCR analysis shows silencing of pluripotency markers ( Sox2 and Oct4 ) and upregulation of the endoderm marker Gata6 in the Spen rescue clones (Supplementary Fig. 3g ), indicating that Spen overexpression does not cause a differentiation phenotype. Interestingly, in undifferentiated Spen −/−(cDNA) ESC clones, Xist levels were higher than in Wt controls (Fig. 2a ), and Xist RNA-FISH analysis revealed a significant percentage of Spen −/−(cDNA) undifferentiated ESCs having Xist clouds (Fig. 2b, c ), probably due to higher SPEN abundance after overexpression in the undifferentiated state (Supplementary Fig. 3c ). Fig. 2: Spen cDNA expression in Spen −/− ESCs rescues Xist expression. a Relative total Xist expression determined by RT-qPCR at days 0, 3, and 5 of monolayer differentiation of Wt, Spe n −/− and three independent rescue clones (Clone A, B and C). Average expression ± SD, n = 4 biological replicates per condition. Reference gene: Hist2h2aa1 . b RNA FISH of Xist (red) at days 0 and 3 of monolayer differentiation of Wt, Spen −/− , and Spen rescue clones. DNA stained with DAPI (blue). Scale bar: 10 µm. c Quantification of ( b ), showing the percentage of nuclei with Xist clouds in each condition. Average percentage, n = 2 biological replicates, the total number of counted nuclei is indicated. Full size image SPEN accumulation on the Xi early during XCI In light of the previous results, we expect SPEN to accumulate on the Xi at the very early steps of physiological XCI. To investigate this hypothesis and since commercial SPEN antibodies suitable for immunofluorescence (IF) are lacking, we generated ESCs endogenously expressing a C-terminally tagged SPEN-GFP (Supplementary Fig. 4a ). Correct GFP integration was confirmed by PCR on gDNA and by FACS analysis (Supplementary Fig. 4b,c ). IF detection of GFP at different time points of monolayer differentiation revealed SPEN accumulation as early as day 1 in about 30% of the nuclei (Fig. 3a, b ). This percentage remained stable until day 3, while from day 5 onward, SPEN accumulation increased to plateau at day 7. Interestingly, the intensity of SPEN-GFP accumulations gradually rises as differentiation progresses (Fig. 3c ), suggesting that the number of SPEN molecules increases over time. Fig. 3: SPEN colocalizes with the Xi chromosome very early during monolayer differentiation. a SPEN-GFP IF staining (αGFP, green) at different time points of monolayer differentiation (day 0, 1, 2, 3, 5, 7, 10, and 12). DNA is stained with DAPI (blue). Scale bar: 10 µm. b Quantification of ( a ), depicting the percentage of SPEN-GFP accumulation per nuclei at different time points of monolayer differentiation. Average percentage, n = 2 independent clones, the total number of counted nuclei per clone is indicated. c Boxplots illustrating the intensity of SPEN-GFP accumulations at different days of monolayer differentiation. The box plots display the median (central black line), the interquartile range (box limits) and the whiskers represent 1.5x of the interquartile range. All the data points are shown for two independent SPEN-GFP clones (filled circles vs. crosses). Two-sided Mann–Whitney test corrected with Benjamini–Hochberg for multiple testing ( α < 0.05). The total number of studied nuclei per clone is indicated. d IF (αGFP, green) combined with Xist RNA FISH (red) of SPEN-GFP lines at days 0, 2, and 5 of monolayer differentiation. DNA is stained with DAPI (blue). Scale bar: 10 µm. e Percentage of nuclei with a Xist cloud that also presents SPEN accumulation. Average percentage, n = 2 independent clones, the total number of counted nuclei per clone is indicated. Calculated from the same data as for Supplementary Fig. 4d . f Percentage of nuclei with SPEN accumulation that also present EZH2 or H3K27me3 accumulation. Average percentage, n = 2 independent clones, the total number of counted nuclei per clone is indicated. Calculated from the same data as for Supplementary Fig. 4g . Full size image Previous studies have shown that SPEN and Xist colocalize in doxycycline-inducible Xist undifferentiated ESC lines [20] , [25] , although the normal timing and relationship between SPEN and Xist in differentiating cells remained unexplored. Therefore, we investigated SPEN accumulation in relation to Xist , by performing GFP IF combined with Xist RNA FISH in differentiating cells (Fig. 3d , Supplementary Fig. 4d ). This analysis indicated that at day 2 of differentiation, about 55% of the cells with Xist clouds showed SPEN colocalization (Fig. 3e ). We also studied the relation of SPEN with other key players in XCI, including the PRC2 catalytic subunit EZH2 and its catalytic product H3K27me3. As found for Xist , we could detect colocalization of EZH2 and its associated histone modification with SPEN (Supplementary Fig. 4e–g ). At day 2 of differentiation, about 70% of nuclei with SPEN accumulation displayed EZH2 and 20% H3K27me3 accumulation. At day 5, the percentage of nuclei with SPEN accumulation that also have EZH2 or H3K27me3 is of approximately 80% and 90%, respectively (Fig. 3f ). Our results show that SPEN accumulation on the Xi happens very early upon differentiation in a progressive manner. Xist RNA stability is compromised in Spen −/− ESCs We have shown that SPEN is required for endogenous Xist upregulation and XCI upon ESC differentiation. In addition, we noticed that forced Xist upregulation resulted in reduced Xist RNA levels in Spen −/− cells compared with Wt cells (Fig. 1d , Fig. 4a ). Accordingly, the percentage of nuclei with Xist clouds was lower in Spen −/− cells with doxycycline-induced Xist versus Wt cells and Xist clouds were in general smaller (Fig. 4b, c ), an effect that could be attributed to affected stability of Xist . To study the role of SPEN in Xist stability, we determined the half-life of doxycycline-induced Xist RNA in Spen −/− and Wt ESCs treated with actinomycin D to block its transcription. The remaining levels of Xist RNA at different time points were assessed by RT-qPCR, and the Xist RNA-decay rate and half-life were then calculated (Fig. 4d ). In Wt ESCs, the Xist RNA half-life was 10 h 17 min, whereas the Xist half-life was reduced to 4 h 40 min in Spen −/− cells. These results indicate that SPEN plays a role in Xist RNA stability, but cannot explain why physiological Xist upregulation is lost in Spen −/− ESCs upon differentiation. Fig. 4: SPEN plays a role in Xist RNA stability. a Relative total Xist expression in undifferentiated Wt and Spen −/− ESCs upon Xist induction with doxycycline for 4 days. n = 3 biological replicates per condition. Average expression ± SD. Reference gene: Beta - actin . b Xist RNA FISH (red) of undifferentiated Wt and Spen −/− ESCs treated with doxycycline to induce Xist expression. DNA is stained with DAPI (blue). Scale bar: 10 µm. c Quantification of ( b ), displaying the percentage of nuclei with Xist clouds. Average percentage, n = 2 biological replicates per condition, the total number of counted nuclei is indicated. d Percentage of Xist RNA remaining at different time points of actinomycin D treatment ( t = 0, 2, 6 and 10 h) in undifferentiated Wt and Spen −/− ESCs treated with doxycycline. Normalized relative expression to t = 0 ± SD, shading represents the SD, n = 3 biological replicates per condition. Reference gene: Beta - actin . Full size image SPEN, HDAC3, and H3K27ac are enriched at the Tsix regulatory region Our results showed that at late days of monolayer differentiation, Spen −/− cells display higher Tsix levels than control cells (Fig. 1i ), suggesting that SPEN might be recruited by Xist to silence Tsix . Hence, we explored SPEN genomic binding at the Xist–Tsix locus using published SPEN CUT&RUN data in undifferentiated ESCs with a doxycycline-responsive Xist promoter [25] . SPEN accumulation is evident on the gene body of Xist as well as on the Tsix regulatory region at 24 h of doxycycline induction, but more prominently after 4 and 8 h of induction (Fig. 5a, b ). This Tsix regulatory region comprises the minor and major Tsix promoters and Xite , an enhancer of Tsix [28] . Xist- mediated recruitment of SPEN is important for recruitment and/or activation of HDAC3, responsible for the removal of H3K27ac from the future Xi [16] , [29] . Analysis of published HDAC3 and H3K27ac ChIP-seq data from undifferentiated female ESCs upon 24 h of Xist induction [29] reveals HDAC3 binding and H3K27ac loss at the Tsix regulatory region, where SPEN is recruited (Fig. 5a ). Moreover, X-linked Rnf12 (Supplementary Fig. 5a ) and Pgk1 (Supplementary Fig. 5b ) display SPEN and HDAC3 enrichment at their promoters and H3K27ac loss upon Xist induction. Interestingly, Rnf12 , an early silenced gene [30] , shows SPEN and HDAC3 promoter binding in the undifferentiated state without Xist induction, suggesting that in the undifferentiated state, Xist might be sufficiently expressed at very low levels to partly silence Rnf12 , explaining the Rnf12 allelic ratio difference between Wt and Spen −/− ESCs at day 0 (Fig. 1e , Supplementary Fig. 3e ). Fig. 5: Tsix -regulatory region shows SPEN, HDAC3 and H3K27ac enrichment. a Genome browser tracks showing allele-specific SPEN, HDAC3, H3K27ac and H3K27me3 binding at the Xist – Tsix locus. The top part (dark) of each track represents the Xi and the bottom (light) the Xa. SPEN CUT&RUN (blue, top) profile in Xist- inducible undifferentiated ESCs (day 0) untreated or treated with doxycycline (24 h) [25] . HDAC3 (green, middle–top) and H3K27ac ChIP-seq (yellow, middle–bottom) in Xist- inducible undifferentiated ESC (day 0) untreated or treated with doxycycline (24 h) [29] . H3K27me3 ChIP-seq (red, bottom) in Wt and Spen −/− ESCs at days 0 and 3 of monolayer differentiation. The light-blue rectangle highlights the Tsix regulatory region, including the Tsix minor and major promoters, and Xite . The light-gray rectangle highlights the H3K27me3 hotspot region. The dashed rectangle indicates the genomic region in (b). b Zoom-in view of the Tsix promoter region, showing the SPEN CUT&RUN profile in undifferentiated ESCs (day 0) untreated or treated (4 h, 8 h and 24 h) with doxycycline. Full size image To test whether SPEN recruitment leads to H3K27me3 accumulation, we performed H3K27me3 ChIP-seq on Spen −/− and Wt ESCs prior to and during differentiation (day 3) (Fig. 5a ). This analysis showed that while Wt cells display H3K27me3 enrichment at the Tsix -regulatory region upon differentiation, Spen −/− cells do not, in accordance with their lack of Xist upregulation. Interestingly, the H3K27me3 hotspot, located at the 3′ end of Tsix [31] , [32] , is clearly reduced upon differentiation both in Wt and Spen −/− cells, while Wt and Spen −/− ESCs show no difference in H3K27me3 levels, pointing to a SPEN-independent H3K27me3 enrichment at the hotspot (Fig. 5a ). Altogether, these data support a model where Xist- mediated SPEN recruitment leads to Tsix promoter silencing. SPEN is required to silence Tsix to allow Xist upregulation To further investigate the role of SPEN in silencing Tsix , we generated compound Spen −/− : Tsix -defective hybrid ESC lines. If Xist -mediated recruitment of SPEN to the Tsix regulatory region is crucial for Tsix silencing and Xist upregulation, we expect Xist upregulation upon differentiation to be rescued in these double-knockout cell lines. We made use of a Tsix- Stop line containing a triple poly(A) signal downstream of the major Tsix promoter that blocks its transcription on the 129 allele [7] , and a Tsix- Cherry line with a mCherry coding sequence introduced downstream of the major Tsix promoter on the Cast allele [33] (Fig. 6a ). As controls, we generated Spen −/− ESCs in the same hybrid background (F1:129/Cast) where both Xist alleles are intact [34] , in contrast to the previously studied ESCs that contained a doxycycline-inducible Xist allele. Deletion of the Spen ORF was confirmed in all cell lines by PCR on gDNA and Western blot analysis (Supplementary Fig. 6a,b ). We generated two independent knockout clones per line. All ESC lines were differentiated in biological quadruplicates, followed by allele-specific Xist RNA expression analysis by RT-qPCR. As expected, the F1:129/Cast control Spen −/− line showed no Xist upregulation (Fig. 6b ), similar to the phenotype observed in the Spen knockout clones generated in the heterozygous doxycycline-inducible Xist cell line (Fig. 1f ). Remarkably, the introduction of a poly(A) signal in Spen −/− : Tsix- Stop lines fully rescued Xist upregulation upon differentiation (Fig. 6c ), indicating that SPEN is required for Xist upregulation via Tsix repression. However, the Spen −/− :Tsix- Cherry lines displayed only mild upregulation of Xist upon differentiation (Fig. 6c ). These differences in the rescue phenotype between Spen −/− :Tsix- Cherry and Spen −/− : Tsix- Stop lines can be explained by the remaining Tsix transcription in the Tsix- Cherry line, which is fully ablated in the Tsix- Stop lines (Supplementary Fig. 6c ). As expected, the Spen −/− : Tsix- Stop lines are not able to silence Rnf12 , despite normal Xist levels in the Tsix- Stop line (Supplementary Fig. 6d ). Moreover, the Spen −/− : Tsix- Stop lines display Xist clouds that were similar in morphology and number compared with Wt F1:129/Cast cells (Fig. 6d, e ). Fig. 6: SPEN is required to silence Tsix , to allow Xist upregulation upon XCI initiation. a Schematic overview of the Tsix- defective ESC lines used to study the role of SPEN in Tsix silencing and Xist upregulation, namely, Wt (F1:129/Cast) (top), Tsix- Stop (middle), and Tsix- Cherry (bottom). The Tsix- Stop line is defective for Tsix in the 129 allele; the Tsix- Cherry line is defective in the Cast allele. Homozygous deletion of Spen was performed in the three lines. b Relative allele-specific Xist expression in Wt and Spen −/− F1:129/Cast ESC lines at different time points of monolayer differentiation. Average expression ± SD, n = 4 biological replicates per condition. Reference gene: Hist2h2aa1 . c Same as in ( b ) for Wt and Spen −/− Tsix- Stop and Tsix- Cherry ESC lines. d Xist RNA FISH (red) at day 3 of monolayer differentiation in F1:129/Cast and Tsix- Stop Wt and Spen −/− ESC lines. DNA is stained with DAPI (blue). Scale bar: 10 µm. e Quantification of ( d ), showing the percentage of nuclei with Xist clouds. Average percentage, n = 2 biological replicates per condition, the total number of counted nuclei is indicated. f Percentage of Xist RNA remaining at different time points of actinomycin D treatment ( t = 0, 2, 4, 6, and 10 h) in differentiating Wt and Spen −/− Tsix- Stop ESCs (day 3). Normalized relative expression to t = 0 ± SD, shading represents the SD, n = 3 biological replicates. Reference gene: Beta - actin . Full size image Using a doxycycline-inducible Xist line, we have shown SPEN’s importance in Xist RNA stability (Fig. 4d ). However, since doxycycline-induced Xist expression is about 10 times higher compared with its endogenous expression upon differentiation (Fig. 1d,f ), we wanted to analyze the SPEN’s role in Xist RNA stability when expressed endogenously. For this, we used Wt: and Spen −/− : Tsix -Stop ESCs at day 3 of monolayer differentiation, where Xist is upregulated from its endogenous promoter (Fig. 6c ). In Wt: Tsix -Stop ESCs, Xist RNA’s half-life was 9 h 42 min, while in S pen −/− : Tsix -Stop ESCs, it was reduced to 2 h 46 min (Fig. 6f ), confirming that SPEN is important for Xist RNA stability, independently of the promoter type and RNA abundance. Taken together, our results indicate an essential role for SPEN in Xist upregulation, mainly via silencing of Tsix , and to a lesser extent by stabilizing Xist RNA. SPEN is therefore not only crucial in X-linked gene silencing but also in the early initiation steps of XCI, playing a role in the feedforward loop leading to Xist activation (Fig. 7 ). Fig. 7: Model of the role of SPEN in XCI. In the undifferentiated state, Tsix transcription represses Xist and Tsix RNA levels are high ( a ). Upon differentiation, at the start of XCI ( b – d ), Xist transcription increases ( b ), the nascent Xist transcripts recruit SPEN that is necessary to silence the Tsix promoter through removal of active H3K27ac marks ( c ). Consequently, the silencing of Tsix allows Xist upregulation and accumulation ( d ). Later, during the establishment phase of XCI, the spreading of SPEN- Xist along the X chromosome allows the silencing of active genes ( e , f ). Moreover, SPEN is also necessary to stabilize Xist RNA ( g ). This model, in addition to previous evidence, proposes that SPEN is not only key in X-linked gene silencing, but also in initiation of XCI. Full size image In this study, we show that SPEN-defective ESCs do not upregulate Xist upon differentiation and study the molecular mechanism behind this observation. To explore the role of SPEN in XCI, various studies used Xist- inducible ESC lines to generate SPEN-knockdown or -knockout cell lines (Supplementary Table 1 ). Forcing Xist expression in ESCs is a powerful way to understand X-linked gene silencing, but is not suitable to investigate the initiation phase of XCI. Studies exploring the role of SPEN in cells undergoing physiological XCI involved Spen knockdown strategies [17] , [20] , therefore, the levels of SPEN might have been sufficient to allow normal Xist upregulation, while showing a defect in X-linked gene silencing. Likewise, our Spen +/− ESC lines show Xist upregulation, but reduced X-linked silencing compared with Wt lines. In agreement with our results, one study reports lower Xist abundance and cloud formation upon forced Xist induction from the endogenous locus in Spen −/− ESCs [27] . Another recent study suggested that Spen −/− ESCs are not able to differentiate upon leukemia inhibitory factor (LIF) removal and differentiation towards neural progenitor cells [35] , while we observe that Spen −/− ESCs display a normal morphology in the undifferentiated state and undergo normal differentiation upon monolayer differentiation. Nevertheless, we observe more cell death of Spen −/− cells compared with Wt cells upon monolayer differentiation, although we consider that this might not be XCI-related since X0 Spen −/− cells also die upon differentiation (data not shown). This observation is probably not surprising since SPEN plays a role in various biological processes as a transcriptional repressor [23] , [24] , [36] . Previous studies performed with doxycycline-inducible Xist lines show that SPEN and Xist colocalize soon after Xist induction [20] , [25] . However, Xist upregulation from a doxycycline-inducible promoter happens at a very different timescale than during physiological XCI. In the present study, we observe that cells with SPEN accumulation are detectable from day 1 of differentiation with their number and intensity levels of these accumulations increasing over time, suggesting that SPEN accumulates in a progressive manner. In addition, we provide evidence that SPEN is required to silence Tsix to allow Xist upregulation. (I) In Spen −/− cells, we detect higher levels of Tsix in differentiating cells from the allele undergoing X-chromosome inactivation, compared with Wt cells. In line with this, paternal Tsix levels in female E3.5 blastocysts with a mutated Xist RepA, necessary for SPEN recruitment, are higher than in Wt blastocysts [37] , which is suggestive of defective Tsix silencing in the absence of SPEN. (II) SPEN overexpression in ESCs leads to higher Xist levels and ectopic Xist cloud formation in the undifferentiated state, suggesting that SPEN overexpression might lead to partial silencing of the Tsix promoter, facilitating Xist expression. (III) SPEN binds to active promoters and enhancers to silence the X chromosome [25] . Spatial proximity to the Xist locus is a strong predictor of X-linked gene silencing efficiency [26] , [38] . One of the closest actively transcribed promoters to Xist is Tsix and we indeed observe SPEN binding at the Tsix regulatory region. (IV) Spen −/− cell lines cannot upregulate Xist , while compound Spen : Tsix defective cell lines ( Spen −/− : Tsix -Stop) display normal Xist levels upon differentiation, indicating that in the absence of SPEN, Tsix , which acts as a brake on Xist transcription, cannot be silenced. Furthermore, our results show that SPEN plays a role in Xist stability, both upon forced Xist upregulation in undifferentiated ESCs and in differentiating Tsix -Stop ESCs, in line with a recently published study, where a role for SPEN in RNA Xist stability is described using microscopy-based approaches [39] . During initiation of XCI, when Xist starts to be transcribed from the future Xi, SPEN helps remodel the chromatin environment of the Xist–Tsix locus. SPEN and HDAC3 are present at the Tsix regulatory region and H3K27ac levels decrease upon Xist induction. Accordingly, we propose that during XCI initiation, SPEN binds Xist nascent transcripts [25] , recruits and/or activates HDAC3 [16] , [29] , which removes histone acetylation marks, weakening the Tsix promoter activity and facilitating Xist expression. Then, Xist spreads together with SPEN along the X-chromosome to silence active genes. Moreover, SPEN is necessary for Xist RNA stabilization (Fig. 7 ). The mechanism driving the symmetry breaking event leading to monoallelic upregulation of Xist has been a focus of many studies. Several studies showed that the Xic and more specifically the Xist - Tsix master switch are tightly regulated in a deterministic process, involving monoallelic downregulation of Tsix or X-pairing mechanisms [40] , [41] , [42] . In contrast, our studies, and studies of others, indicate that a gene regulatory network composed of transacting activators and inhibitors of XCI, involving positive- and negative-feedback loops, instructs the cis -regulatory landscape of the Xic to direct monoallelic upregulation of Xist [12] , [34] , [43] , [44] . Tsix silencing not only involves downregulation of inhibitors of XCI, including pluripotency factors OCT4, SOX2, KLF4, c-MYC, and REX1 [45] , [46] , [47] , but also involves Xist- mediated recruitment of SPEN as our present work reveals. This can happen on either allele, but asynchronous Xist transcription bursts will facilitate Xist -mediated monoallelic silencing of Tsix through SPEN, resulting in further upregulation of Xist and concomitant silencing of the XCI activator Rnf12 , providing a negative feedback loop to prevent upregulation of Xist on the future active X chromosome. In humans, SPEN seems to play a role in XCI [48] even though in-depth mechanistic studies are missing, but whether SPEN is required for XIST upregulation is unknown. In addition, TSIX does not completely overlap XIST and does not seem to be a strong regulator of XIST [49] , [50] , therefore, a mechanism in which SPEN negatively regulates TSIX to allow XIST upregulation is not very likely. However, the possibility that SPEN controls other human-specific XIST regulators should be taken into consideration. Cell culture Mouse ESCs were grown on feeder cells, Wt C57BL/6 male-irradiated mouse embryonic fibroblasts (MEFs), and medium containing DMEM (Gibco, 11995065), 15% fetal calf serum (FCS) (Capricorn Scientific, FBS-12A), 0.1 mM nonessential amino acids (NEAA) (Lonza, BE13-114E), 100 U mL −1 penicillin, 100 ug mL −1 streptomycin (Sigma-Aldrich, P0781), 0.1 mM 2-mercaptoethanol (Gibco, 31350010) and 5.000 U mL −1 LIF. Previous to monolayer differentiation cells were plated in nongelatinized plates to eliminate feeder cells. Then, plated at specific densities per time point in differentiation medium composed of IMDM-glutamax (Gibco, 31980030), 15% FCS, 0.1 mM NEAA, 100 U mL −1 penicillin, 100 µg mL −1 streptomycin, 37.8 µL L −1 monothioglycerol (Sigma-Aldrich, M6145) and 50 µg mL −1 ascorbic acid (Sigma-Aldrich, A92902). When appropriate, the medium was supplemented with 2 μg mL −1 doxycycline (Sigma-Aldrich, D9891). 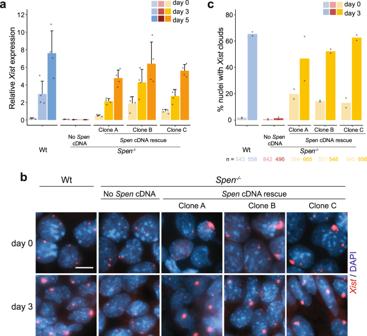Fig. 2:SpencDNA expression inSpen−/−ESCs rescuesXistexpression. aRelative totalXistexpression determined by RT-qPCR at days 0, 3, and 5 of monolayer differentiation of Wt,Spen−/−and three independent rescue clones (Clone A, B and C). Average expression ± SD,n= 4 biological replicates per condition. Reference gene:Hist2h2aa1.bRNA FISH ofXist(red) at days 0 and 3 of monolayer differentiation of Wt,Spen−/−, andSpenrescue clones. DNA stained with DAPI (blue). Scale bar: 10 µm.cQuantification of (b), showing the percentage of nuclei withXistclouds in each condition. Average percentage,n= 2 biological replicates, the total number of counted nuclei is indicated. Gene editing using the CRISPR/Cas9 technology Different female F1 2–1 hybrid (129/Sv-Cast/Ei) ESC lines with different genetic modifications to interrogate various aspects of XCI were targeted in this study (Supplementary Table 2 ). To generate Spen heterozygous and homozygous knockout clones two single-guide RNAs (sgRNA) targeting the 5′ (5′-AGTGCGCTTCGTCACTGCAC-3′) and 3′ (5′-TCCTCCCGCCCCGACGCGGA-3′) region of the Spen ORF were cloned in the Cas9-GFP pX458 vector (Addgene plasmid #48138). Compatible 5′ and 3′ homology arms (HA) of approximately 500 bp were amplified by PCR from mouse gDNA and cloned in the pCR-Blunt-II-TOPO vector with a NdeI restriction site in-between the 5′ and 3′ HA. This site was used to insert a puromycin resistance (PuroR) cassette flanked by loxP sites. The ROSA26 locus was targeted using the pX458 vector coding for a sgRNA (5′-CGCCCATCTTCTAGAAAGAC-3′) compatible with the pFD46 expression vector [25] , coding for the Spen cDNA and a hygromycin resistance cassette. To create an endogenous Spen C-terminal enhanced GFP (eGFP) knock-in, a sgRNA targeting the 3′ end of Spen ORF (5′-ATTGTCATTGCCTCGGTGTG-3′) was cloned in the Cas9-PuroR pX459 vector (Addgene plasmid #62988). The donor template was made using a gblock from Integrated DNA Technologies coding for compatible 5′ and 3′ HA of 600 bp with a NheI and AscI restrictions sites in-between the 5′ and 3′ HA, which were used to insert an eGFP in frame with the Spen coding sequence. To clone the sgRNAs, two complementary oligonucleotides coding for the desired target sequence and overhangs compatible with the restriction enzyme BsbI were annealed and ligated in the pX458 or px459 plasmids, that were previously digested with BsbI. The appropriate plasmid combinations were transfected into ESCs using Lipofectamine 2.000 (Invitrogen, 11668019) and plated at low density to obtain single colonies, when the appropriate medium was supplemented with 1 µg mL −1 puromycin (Sigma-Aldrich, P8833) for 48–72 h or 250 μg mL −1 hygromycin B (Invitrogen, 10687010) for 7 days. 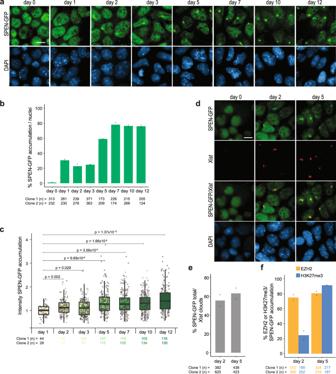Fig. 3: SPEN colocalizes with the Xi chromosome very early during monolayer differentiation. aSPEN-GFP IF staining (αGFP, green) at different time points of monolayer differentiation (day 0, 1, 2, 3, 5, 7, 10, and 12). DNA is stained with DAPI (blue). Scale bar: 10 µm.bQuantification of (a), depicting the percentage of SPEN-GFP accumulation per nuclei at different time points of monolayer differentiation. Average percentage,n= 2 independent clones, the total number of counted nuclei per clone is indicated.cBoxplots illustrating the intensity of SPEN-GFP accumulations at different days of monolayer differentiation. The box plots display the median (central black line), the interquartile range (box limits) and the whiskers represent 1.5x of the interquartile range. All the data points are shown for two independent SPEN-GFP clones (filled circles vs. crosses). Two-sided Mann–Whitney test corrected with Benjamini–Hochberg for multiple testing (α< 0.05). The total number of studied nuclei per clone is indicated.dIF (αGFP, green) combined withXistRNA FISH (red) of SPEN-GFP lines at days 0, 2, and 5 of monolayer differentiation. DNA is stained with DAPI (blue). Scale bar: 10 µm.ePercentage of nuclei with aXistcloud that also presents SPEN accumulation. Average percentage,n= 2 independent clones, the total number of counted nuclei per clone is indicated. Calculated from the same data as for Supplementary Fig.4d.fPercentage of nuclei with SPEN accumulation that also present EZH2 or H3K27me3 accumulation. Average percentage,n= 2 independent clones, the total number of counted nuclei per clone is indicated. Calculated from the same data as for Supplementary Fig.4g. Colonies were screened by PCR for correct integration of the desired construct (Supplementary Table 3 ). Positive clones were further characterized by Western blot, RT-qPCR and/or FACS, and the presence of 2 X chromosomes and correct karyotype was also assessed. Full scan images of all the genotyping gels are available in the Source Data file. Protein extraction and Western blot To prepare nuclear extracts all procedures were done at 4 o C and buffers supplemented with 1x protease inhibitors (Roche, 4693132001), 15 µM MG-132 (Sigma-Aldrich, C2211) and 0.5 mM DTT. Cells were harvested by scraping in cold PBS, collected and centrifuged (200 × g , 5 min, 4°C). The pellet was incubated in 5x the pellet volume of Buffer A (10 mM Hepes pH 7.6, 1.5 mM MgCl 2 , and 10 mM KCl) for 10 min, vortexed (30 sec) and centrifuged (900 × g , 5 min, 4°C). Then, the pellet was resuspended in 1.5x Buffer C (20 mM Hepes pH 7.6, 25% glycerol, 420 mM NaCl, 1.5 mM MgCl 2 , and 0.2 mM EDTA) and rotated (30 min, 4°C). The solution was centrifuged (18,000 × g , 10 min, 4°C) and the supernatant collected as nuclear extract. The protein concentration was measured using Nanodrop and all samples diluted to the same concentration using Buffer C. NuPAGE™ LDS Sample Buffer (4X) (Invitrogen, NP0007) containing 5% b-mercaptoethanol was added to nuclear extracts, and boiled (95°C, 5 min). For Western blot analysis, the NuPAGE™ 3–8% Tris-Acetate gels (Invitrogen, EA03755) were used with Tris-Acetate SDS Running Buffer (pH 8.24) (Invitrogen, LA0041) and the HiMark Pre-Stained Protein Standard (Invitrogen, LC5699). Wet transfer on a PVDF membrane was done overnight at 40 mA, with the NuPAGE™ Transfer Buffer (Invitrogen, NP00061), containing 10% methanol and 0.1% SDS. After blocking, the membrane was incubated with the appropriate primary antibodies, SPEN antibody (Abcam, ab72266, 1:2.000), Anti-Flag antibody M2-Peroxidase (Sigma-Aldrich, A8592, 1:3.000) and/or VCP antibody (Abcam, ab11433, 1:20.000), and appropriate secondary antibodies, IRDye 800CW donkey-anti-rabbit (LI-COR Biosciences, P/N 925-32213, 1:10.000), IRDye 680RD donkey-anti-mouse (LI-COR Biosciences, P/N 925-68072, 1:15.000) and/or Goat anti-mouse–Peroxidase antibody (Sigma-Aldrich, A4416, 1:4.000). Full scan images of all the Western blots are available in the Source Data file. RT-qPCR Total RNA was isolated from cell pellets using the ReliaPrep RNA Cell Miniprep System (Promega, Z6012) and reversed-transcribed using Superscript III (Invitrogen, 18080093) and random hexamers (Invitrogen, N8080127), following the manufacturer’s instructions. All RT-qPCRs were done using the GoTaq qPCR Master Mix (Promega, A6002) in a CFX384 real-time PCR-detection system (Bio-Rad). Hist2h2aa1 was used as a normalization control, except in the RNA-stability assays where Beta-actin was used. 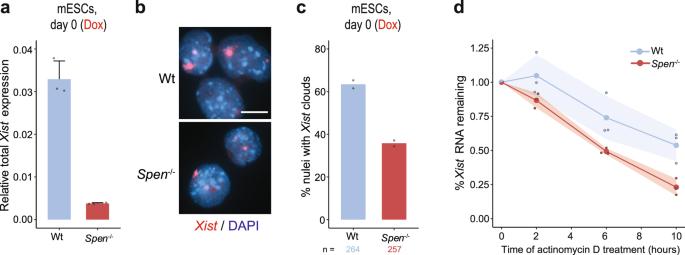Fig. 4: SPEN plays a role inXistRNA stability. aRelative totalXistexpression in undifferentiated Wt andSpen−/−ESCs uponXistinduction with doxycycline for 4 days.n= 3 biological replicates per condition. Average expression ± SD. Reference gene:Beta-actin.bXistRNA FISH (red) of undifferentiated Wt andSpen−/−ESCs treated with doxycycline to induceXistexpression. DNA is stained with DAPI (blue). Scale bar: 10 µm.cQuantification of (b), displaying the percentage of nuclei withXistclouds. Average percentage,n= 2 biological replicates per condition, the total number of counted nuclei is indicated.dPercentage ofXistRNA remaining at different time points of actinomycin D treatment (t= 0, 2, 6 and 10 h) in undifferentiated Wt andSpen−/−ESCs treated with doxycycline. Normalized relative expression tot= 0 ± SD, shading represents the SD,n= 3 biological replicates per condition. Reference gene:Beta-actin. All expression primers are listed in Supplementary Table 4 . The optimal allele-specific primer-pair concentration to amplify the 129 and Cast allele at the same efficiency was optimized using pure 129, Cast and 129-Cast gDNA. RNA-stability assay To study the Xist RNA stability in undifferentiated ESCs, Wt and Spen −/− ESC lines with a doxycycline-responsive Xist promoter were cultured in ESC medium supplemented with doxycycline to induce Xist expression for four days. While in doxycycline treatment, 5 µg mL −1 actinomycin D (Sigma-Aldrich, A1410) was added for different time ( t = 0, 2, 6, and 10 h). Before collection, ESCs were plated in nongelatinized plates to remove the feeders. To study the Xist RNA stability in differentiating Wt and Spen −/− Tsix -Stop ESCs, cells were differentiated, as explained in the “Cell culture” methods section, and 5 µg mL -1 actinomycin D were added for different time ( t = 0, 2, 4, 6, and 10 h). In both cases, cells were harvested for RNA isolation, cDNA synthesis and RT-qPCR. 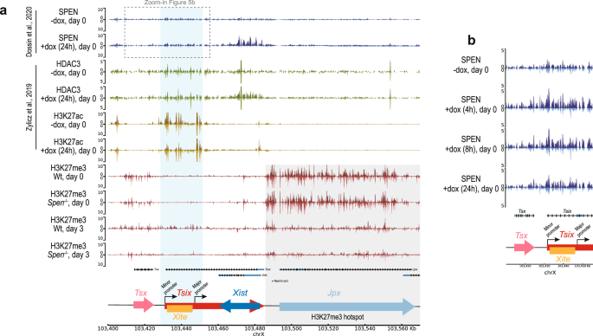Fig. 5:Tsix-regulatory region shows SPEN, HDAC3 and H3K27ac enrichment. aGenome browser tracks showing allele-specific SPEN, HDAC3, H3K27ac and H3K27me3 binding at theXist–Tsixlocus. The top part (dark) of each track represents the Xi and the bottom (light) the Xa. SPEN CUT&RUN (blue, top) profile inXist-inducible undifferentiated ESCs (day 0) untreated or treated with doxycycline (24 h)25. HDAC3 (green, middle–top) and H3K27ac ChIP-seq (yellow, middle–bottom) inXist-inducible undifferentiated ESC (day 0) untreated or treated with doxycycline (24 h)29. H3K27me3 ChIP-seq (red, bottom) in Wt andSpen−/−ESCs at days 0 and 3 of monolayer differentiation. The light-blue rectangle highlights theTsixregulatory region, including theTsixminor and major promoters, andXite. The light-gray rectangle highlights the H3K27me3 hotspot region. The dashed rectangle indicates the genomic region in (b).bZoom-in view of theTsixpromoter region, showing the SPEN CUT&RUN profile in undifferentiated ESCs (day 0) untreated or treated (4 h, 8 h and 24 h) with doxycycline. Then, total Xist levels were determined and normalized to Beta-actin and the percentage of the remaining Xist RNA was calculated by dividing Xist expression levels at the different times of collection relative to t = 0. Using linear regression analysis the RNA decay rate constant ( k decay ) was calculated from the slope of the curve that best fitted our data and the RNA half-life ( t 1/2 ) obtained with the following formula \({t}_{1/2}=\frac{{ln}2}{{k\; {{{{{\rm{decay}}}}}}}}\,\) . Immunofluorescence (IF) Undifferentiated ESCs were attached to slides using a cytospin, while differentiating cells were grown on coverslips coated with gelatin (Sigma-Aldrich, G1890) or laminin (Sigma-Aldrich, L2020). Cells were fixed with 4% paraformaldehyde (PFA) in PBS (10 min, RT), permeabilized with 0.4% Triton-X100 and 5% goat serum in PBS (15 min, on ice) and blocked with 10% goat serum in PBST, composed of 0.05% Tween-20 in PBS (30 min, RT). Primary antibody incubation was done in blocking buffer (2 h, RT), after three washings with PBST the slides were incubated with the secondary antibody (1 h, RT). After three washings, the second washing containing DAPI, the slides were mounted with ProLong Gold antifade mounting medium (Invitrogen, P36930). The used primary antibodies were the following: αGFP (Abcam, ab290, 1:500), H3K27me2/3 (Active motif, 39535, 1:100) and EZH2 (BD43 clone, kindly provided by Dr. Kristian Helin, 1:100). The used secondary antibodies were Goat-anti-Rabbit-488 (Invitrogen, A-11008 1:1.000) and Goat-anti-Mouse-546, (Invitrogen, A-1103, 1:400). Images were taken using a ZEISS Axio Imager M2 including digital microscopy camera AxioCam 503 and analyzed with ImageJ. To quantify the intensity of the SPEN-GFP accumulation at different days of monolayer differentiation, we determined the mean intensity of a region of interest (ROI) covering a specific SPEN-GFP accumulation. Next, this value was normalized to the mean nuclei background intensity excluding the SPEN-GFP ROI, calculated as the average intensity of 10 different nuclei per image. IF combined with RNA fluorescent in situ hybridization (FISH) The Xist FISH probe was made from 2 µg of a 5.5 kb DNA fragment of mouse Xist comprising exons 3–7. Fluorescent labeling was done with dUTP SpectrumRed using the nick translation kit (Abbott, 07J00-001) overnight at 16 o C. The probe was purified with ProbeQuant G-50 Micro Columns (GE, GE28-9034-08), combined with 100 µg of mouse tRNA, 20 µg of mouse Cot-1 DNA (Invitrogen, 18440-016) and 100 µg of salmon sperm DNA (Invitrogen, 15632-011) and precipitated with 2 M NaAc (pH 5.6) and 100% EtOH. The pellet was resuspended in 50 µL hybridization mix (50% formamide, 10% dextran sulfate in 2xSSC) and stored at −20°C. Before use, 20 µL of probe was prehybridized (10 min, 75 o C) with 0.5 µg of mouse Cot-1 DNA supplemented with 10 mM vanadyl ribonucleoside complex (VRC) (NEB, S1402S) and 0.2 U µL − 1 RNAseOUT (Invitrogen, 10777019). Cells on coverslips or slides were fixed with 4% PFA in PBS (10 min, RT), permeabilized with 0.5% Triton-X100 in PBS and blocked in TS-BSA buffer (0.1 M Tris-HCl (pH 7.5), 0.15 M NaCl, and 2 mg mL − 1 BSA (Jena Bioscience, BU-102) in H 2 O). The αGFP (Abcam, ab290, 1:500) primary antibody was incubated in blocking buffer (30 min, 37°C), washed in PBS (3x) and then incubated with the secondary antibody (30 min, 37°C). All solutions were supplemented with 10 µM VRC and 0.2 U µL −1 RNAseOUT. Slides were washed in PBS (3x), post-fixed with 4% PFA (10 min, RT), and washed again in PBS (x3). Dehydration was done with increasing ethanol concentrations (70%, 90% and 100%). The prehybridized probe was added on top of the coverslips or slides (20 h, 37 o C, humid chamber). Various washings were done with 50% formamide/2x SSC (5 min, 37 o C, 2x), 2x SSC (5 min, 37 o C, 2x) and TS buffers (5 min, RT, 2x). Then the slides were mounted and visualized as explained in the “IF” section. FISH The FISH only protocol was done as described in the IF-FISH section, skipping the IF section. Directly after the permeabilization, the dehydration step was performed. RNA-seq Doxycycline treated cells were sorted to isolate dsRed positive cells upregulating Xist from the desired allele. 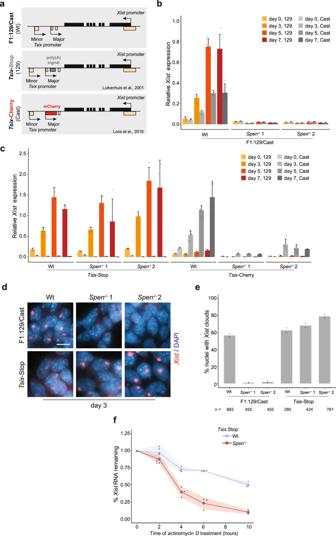Fig. 6: SPEN is required to silenceTsix, to allowXistupregulation upon XCI initiation. aSchematic overview of theTsix-defective ESC lines used to study the role of SPEN inTsixsilencing andXistupregulation, namely, Wt (F1:129/Cast) (top),Tsix-Stop (middle), andTsix-Cherry (bottom). TheTsix-Stop line is defective forTsixin the 129 allele; theTsix-Cherry line is defective in the Cast allele. Homozygous deletion ofSpenwas performed in the three lines.bRelative allele-specificXistexpression in Wt andSpen−/−F1:129/Cast ESC lines at different time points of monolayer differentiation. Average expression ± SD,n= 4 biological replicates per condition. Reference gene:Hist2h2aa1.cSame as in (b) for Wt andSpen−/−Tsix-Stop andTsix-Cherry ESC lines.dXistRNA FISH (red) at day 3 of monolayer differentiation in F1:129/Cast andTsix-Stop Wt andSpen−/−ESC lines. DNA is stained with DAPI (blue). Scale bar: 10 µm.eQuantification of (d), showing the percentage of nuclei withXistclouds. Average percentage,n= 2 biological replicates per condition, the total number of counted nuclei is indicated.fPercentage ofXistRNA remaining at different time points of actinomycin D treatment (t= 0, 2, 4, 6, and 10 h) in differentiating Wt andSpen−/−Tsix-Stop ESCs (day 3). Normalized relative expression to t = 0 ± SD, shading represents the SD,n= 3 biological replicates. Reference gene:Beta-actin. 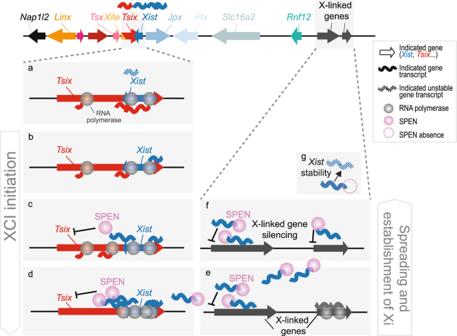Fig. 7: Model of the role of SPEN in XCI. In the undifferentiated state,Tsixtranscription repressesXistandTsixRNA levels are high (a). Upon differentiation, at the start of XCI (b–d),Xisttranscription increases (b), the nascentXisttranscripts recruit SPEN that is necessary to silence theTsixpromoter through removal of active H3K27ac marks (c). Consequently, the silencing ofTsixallowsXistupregulation and accumulation (d). Later, during the establishment phase of XCI, the spreading of SPEN-Xistalong the X chromosome allows the silencing of active genes (e,f). Moreover, SPEN is also necessary to stabilizeXistRNA (g). This model, in addition to previous evidence, proposes that SPEN is not only key in X-linked gene silencing, but also in initiation of XCI. RNA was isolated using the ReliaPrep RNA Cell Miniprep System. A total of 16 DNA libraries were created, a maximum of 1 ng of total RNA was used following the Smart-seq2 protocol [51] without modifications. Then, we used the Nextera DNA Flex library prep kit (Illumina) to create a library from full-length cDNA. Samples were sequenced on a HiSeq2500 sequencer (50 bp single-end reads). Chromatin immunoprecipitation (ChIP)-seq In total, 50 × 10 6 cells were trypsinized, resuspended and fixed in 50 mL of warm medium and 1% PFA for 10 min at 37 o C. About 2.5 mL of Glycine 2.5 M were added to the cells (final concentration 0.125 M) to quench the PFA, 5 min RT on a rotator. All buffers from now on contain protease inhibitors (Roche, 4693132001). Cells were washed twice with cold PBS. Then 1x in 10 mL of Buffer 1 (10 mM Hepes pH 7.5, 10 mM EDTA, 0.5 mM EGTA, and 0.75% Triton X-100) and 1x in Buffer 2 (10 mM Hepes pH 7.5, 200 mM NaCl, 1 mM EDTA, 0.5 mM EGTA), 10 min rotating at 4 o C. Nuclei were then resuspended in Lysis/Sonication Buffer (150 mM NaCl, 25 mM Tris-HCl pH 7.5, 5 mM EDTA, 1% Triton, 0.1% SDS, 0.5% Sodium deoxycholate) and incubated for 30 min on ice. Nuclei were then sonicated 2 × 15 min (30′′ ON/OFF, max input, ice cold water) in a Bioruptor. A small fraction of the lysate was run on a gel to confirm size population of 100–500 bp. About 1 µg of H3K27me3 antibody (Cell Signaling, 9733 S) was conjugated with 25 µL of magnetic beads (Life Technologies, 10004D) for 3 h rotating at 4°C. About 25 ug of chromatin was IP’d with the Ab-beads overnight rotating at 4°C. Beads were washed 2x in standard RIPA buffer (140 mM NaCl, 10 mM Tris-HCl pH 7.5150 mM NaCl, 1 mM EDTA pH8.0, 0.5 mM EGTA pH 8.0, 1% Triton, 0.1% SDS, 0.5% Sodium deoxycholate), and 1x in High Salt RIPA (same as standard RIPA but with 500 mM NaCl), 1x LiCl RIPA (same as standard RIPA but with 250 mM LiCl instead of NaCl) and rinsed once with TE, 10 min 4°C each wash. Chromatin was eluted with 450 µL of Elution Buffer (1% SDS; 0.1 M NaHCO 3 in H 2 O) with 22 µL protease K (10 mg mL −1 ) and 5 µL RNAse A (10 mg mL −1 ) and shaken at 1,000 rpm on an orbital thermal-mixer for 2 h at 37°C first and then 65 o C overnight. DNA was then Phenol–Chloroform extracted and resuspended in 20 µL of H 2 O. About 0.25 µL was used per PCR to confirm the ChIP’s success. The concentration was then measured and a ChIP-seq library was prepared using the ThruPLEX DNA-Seq Kit (Takara Bio, R400675), by following the manufacturer’s instructions: template preparation to obtain a homogeneous double-stranded DNA material, library synthesis to ligate stem-loop adapters and a final library amplification step to extend the template, remove the stem-loop adapters and amplify the library for posterior sequencing on an Illumina HiSeq 2500 sequencer (50 bp paired-end reads). NGS data analysis: allele-specific RNA-seq and ChIP-seq Both the RNA-seq and the ChIP-seq data were processed allele-specifically. The single nucleotide polymorphism (SNPs) in the 129/Sv and Cast/Ei lines was downloaded from the Sanger institute (v.5 SNP142) [52] . These were used as input for SNPsplit v0.3.4 [53] , to construct an N-masked reference genome based on mm10 in which all SNPs between 129/Sv and Cast/Ei were masked. The 50 bp single-end RNA-seq and 50 bp paired-end ChIP-seq reads were mapped to this N-masked reference genome using the default settings of hisat2 v2.2.1 and bowtie2 v2.4.1, respectively [54] , [55] . SNPsplit (--paired for the ChIP-seq analysis) was then used to assign the reads to either the 129/Sv or Cast/Ei bam file based on the best alignment or to a common bam file if mapping to a region without allele-specific SNPs. The allele-specific and unassigned bam files were sorted using samtools v1.10 [56] . For the RNA-seq, the number of mapped reads per gene were counted for both alleles separately using HTSeq v0.12.4 (--nonunique=none -m intersection-nonempty) [57] based on the gene annotation from ensembl v98. For each condition, genes with more than 20 allele-specific reads across both replicates were used to calculate the allelic ratio, defined as \(\left(\frac{{Xi}}{{Xi}+{Xa}}\right).\) For day 0 and day 7, Cast/Ei and 129/Sv were used as the Xi and active allele (Xa), respectively, whereas for day 3, Cast/Ei and 129/Sv were used as Xa and Xi, respectively. The allelic ratios of X-linked genes were visualized as violin plots with boxplots of the same data on top. Significant differences between conditions were tested using a two-sided Mann–Whitney test with α < 0.05. P-values were corrected for multiple testing using the Benjamini–Hochberg procedure. Different conditions were compared by plotting the X-linked genes that had more than 20 allele-specific reads in both conditions along the X chromosome. A two-sided Wilcoxon signed-rank test with α < 0.05 was used to test for significant differences between the allelic ratios of the different conditions, after which P-values were corrected for multiple testing using the Benjamini–Hochberg procedure. We visualized differences in allelic ratios of X-linked genes between conditions by plotting both ratios on the different axes of a scatter plot. Genes were highlighted when they were identified as lowly silenced genes in Spen −/− ESCs from [27] , which were defined as genes showing −0.05 < z < -0.2 where z (gene silencing) = \(\left(\frac{{Xi}}{{Xi}+{Xa}}\right){dox}-\left(\frac{{Xi}}{{Xi}+{Xa}}\right){noDox}\) . The allele-specific ChIP-seq bam files were normalized using the ‘callpeak’ and ‘bdgcmp’ functions of MACS2 v2.2.7.1 [58] . We called broad peaks (-f BAMPE --broad --bdg) and used the Poisson P-value as the method for normalizing the tracks. The input-normalized tracks were visualized using pyGenomeTracks v3.4. [59] . For validation, we downloaded several publicly available datasets. The SPEN CUT&RUN data ( GSE131782 , samples: SRX5903674, SRX5903675, SRX5903676, SRX5903677, SRX5903678, SRX5903679, SRX5903682, and SRX5903683) [25] , were processed similar to our analysis using a C57BL/6NJ-Cast/Ei reference genome. However, the allele-specific tracks were normalized based on the total number of mapped reads per sample. The scaling factor was calculated as 10^6 / total number of mapped reads and used as parameter --scaleFactor to both allelic tracks using deepTools bamCoverage v3.5.0. [60] . A binsize of 1 was used and paired-end reads were extended. The allele-specific tracks from HDAC3 and H3K27Ac ( GSE116990 , samples: SRX4384412, SRX4384420, SRX4384476, SRX4384484, SRX4887836, and SRX4887839) were downloaded from [29] . For all datasets, replicates for each condition were averaged using deepTools bigwigCompare v.3.5.0 with the settings ‘--operation mean --binSize 1’ [60] . In the genome browser overview showing the allele-specific tracks, the y axis was scaled for each group of samples separately. Reporting summary Further information on research design is available in the Nature Research Reporting Summary linked to this article.